Chromatin remodelling and antisense-mediated up-regulation of the developmental switch geneeud-1control predatory feeding plasticity Phenotypic plasticity has been suggested to act through developmental switches, but little is known about associated molecular mechanisms. In the nematode Pristionchus pacificus , the sulfatase eud-1 was identified as part of a developmental switch controlling mouth-form plasticity governing a predatory versus bacteriovorous mouth-form decision. Here we show that mutations in the conserved histone-acetyltransferase Ppa-lsy-12 and the methyl-binding-protein Ppa-mbd-2 mimic the eud-1 phenotype, resulting in the absence of one mouth-form. Mutations in both genes cause histone modification defects and reduced eud-1 expression. Surprisingly, Ppa-lsy-12 mutants also result in the down-regulation of an antisense- eud-1 RNA. eud-1 and antisense- eud-1 are co-expressed and further experiments suggest that antisense- eud-1 acts through eud-1 itself. Indeed, overexpression of the antisense- eud-1 RNA increases the eud-1 -sensitive mouth-form and extends eud-1 expression. In contrast, this effect is absent in eud-1 mutants indicating that antisense- eud-1 positively regulates eud-1 . Thus, chromatin remodelling and antisense-mediated up-regulation of eud-1 control feeding plasticity in Pristionchus . Developmental (phenotypic) plasticity has been suggested to facilitate morphological novelty and diversity [1] , [2] , [3] , [4] , [5] , but little is known about the molecular aspects of developmental switch mechanisms that underlie plasticity. The nematode Pristionchus pacificus is a potential model system to study the molecular and mechanistic details of developmental plasticity because it can be easily cultured in the laboratory by feeding on bacteria, but in the wild it lives in a necromenic interaction with beetles [6] , [7] . Specifically, the necromenic life style of P. pacificus and related nematodes is facilitated by dynamic feeding mode switching between bacterial grazing and the predation of other nematodes ( Fig. 1a,b ; ref. 7 ). This feeding diversity relies on the presence of moveable teeth and Pristionchus nematodes exhibit two distinct morphs—stenostomatous (St, narrow-mouthed) or eurystomatous (Eu, wide-mouthed) —that differ in the number and shape of associated teeth and the size and form of the buccal cavity [8] ( Fig. 1c,d ). When fed on Escherichia coli OP50 bacteria under lab conditions, P. pacificus California reference strain RS2333 hermaphrodites have a stable 70:30% Eu:St ratio, but this can be influenced by starvation, crowding and pheromone signalling [8] , [9] , [10] . Because P. pacificus hermaphrodites reproduce primarily by selfing, strains are genetically homogeneous, and the presence of two distinct morphs thus represents an example of developmental plasticity, which was also demonstrated experimentally [8] . 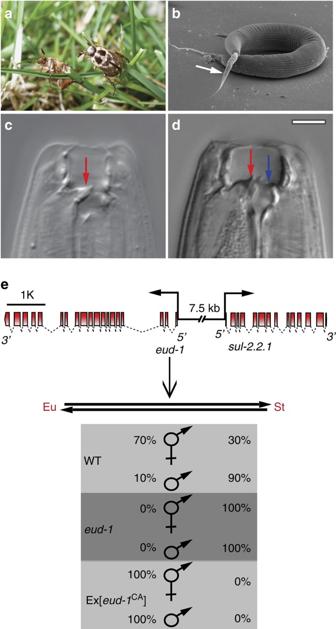Figure 1: Developmental plasticity inP. pacificusand its regulation by the developmental switch geneeud-1. (a) The oriental beetleExomala orientalisis one of the beetle hosts with whichP. pacificuslives in a necromenic association. (b) Scanning electron micrograph showingP. pacificuspredatory feeding on a small larva ofC. elegans(white arrow). (c,d) Mouth dimorphism ofP. pacificusenabling a switch between bacterial grazing and predatory feeding. Stenostomatous (St) animals (c) have a narrow buccal cavity and a flint-like dorsal tooth (red arrow), but miss the subventral tooth. In contrast, eurystomatous (Eu) animals (d) have a wide buccal cavity, a claw-like dorsal tooth (red arrow) and an additional subventral tooth (blue arrow). Scale bars, 10 μm. (e) Molecular organization of theeud-1locus and effect ofeud-1function on mouth-form ratios.eud-1derives from a recent gene duplication, with the neighbouring sulfatasesul-2.2.1arranged in a head-to-head orientation. The two genes are separated by a 7.5 kb intergenic region that when used as promoter drives the expression ofeud-1in various head neurons. In wild-type animals, hermaphrodites and males form∼70% and 10% Eu animals, respectively. Ineud-1mutants, both sexes are completely St, whereaseud-1overexpression causes both genders to form only Eu animals indicating that EUD-1 functions as developmental switch. Figure 1: Developmental plasticity in P. pacificus and its regulation by the developmental switch gene eud-1 . ( a ) The oriental beetle Exomala orientalis is one of the beetle hosts with which P. pacificus lives in a necromenic association. ( b ) Scanning electron micrograph showing P. pacificus predatory feeding on a small larva of C. elegans (white arrow). ( c , d ) Mouth dimorphism of P. pacificus enabling a switch between bacterial grazing and predatory feeding. Stenostomatous (St) animals ( c ) have a narrow buccal cavity and a flint-like dorsal tooth (red arrow), but miss the subventral tooth. In contrast, eurystomatous (Eu) animals ( d ) have a wide buccal cavity, a claw-like dorsal tooth (red arrow) and an additional subventral tooth (blue arrow). Scale bars, 10 μm. ( e ) Molecular organization of the eud-1 locus and effect of eud-1 function on mouth-form ratios. eud-1 derives from a recent gene duplication, with the neighbouring sulfatase sul-2.2.1 arranged in a head-to-head orientation. The two genes are separated by a 7.5 kb intergenic region that when used as promoter drives the expression of eud-1 in various head neurons. In wild-type animals, hermaphrodites and males form ∼ 70% and 10% Eu animals, respectively. In eud-1 mutants, both sexes are completely St, whereas eud-1 overexpression causes both genders to form only Eu animals indicating that EUD-1 functions as developmental switch. Full size image The existence of developmental switch mechanisms is essential for the irreversible control of plasticity and has long been anticipated by evolutionary theory [1] , but associated mechanisms are largely unknown. We have recently identified the sulfatase eud-1 as part of a genetic network that constitutes the developmental switch for the P. pacificus mouth-form decision [6] . In eud-1 mutants, the Eu form is absent ( eud , eu rystomatous-form- d efective), whereas overexpression from transgenes fixes the Eu form, thus confirming that EUD-1 acts as a developmental switch [6] . eud-1 is X-linked and dosage-dependent, and it regulates differences in mouth-form frequency between hermaphrodites and males, among P. pacificus strains, and between Pristionchus species [6] . Interestingly, P. pacificus eud-1 derives from a recent duplication that resulted in two neighbouring gene copies arranged in a head-to-head orientation ( Fig. 1e ). eud-1 is expressed in a small number of P. pacificus head neurons, where its expression is sufficient to induce the execution of the Eu mouth-form [6] . However, while eud-1 expression is highly regulated, the underlying mechanisms that control this developmental switch gene remain unknown. Here we show that mutations in the conserved histone acetyltransferase Ppa-lsy-12 and the methyl-binding-protein Ppa-mbd-2 result in the absence of the Eu mouth-form similar to mutants in Ppa-eud-1 . Mutations in both genes cause histone modification defects that result among others, in reduced eud-1 expression. In addition, in Ppa-lsy-12 mutants an antisense- eud-1 RNA is also down-regulated. Overexpression of the antisense- eud-1 RNA from transgenes increases the eud-1 -sensitive mouth-form and results in increased eud-1 expression. In contrast, this effect is absent in eud-1 mutants indicating that antisense- eud-1 positively regulates eud-1 . These epigenetic mechanisms provide a theoretical framework for linking genetic regulation to environmental input. Two pleiotropic mutants with mouth-form defects To study the regulation of eud-1 , we searched for pleiotropic mutants with a Eud phenotype in hermaphrodites, similar to eud-1 . By screening more than 30 already-established mutant strains with egg laying- or vulva defects, we identified two mutants, tu319 and tu365 , with a nearly complete loss of the Eu form ( Fig. 2a ). While tu319 was previously molecularly uncharacterized, tu365 represents a deletion allele in the methyl-binding protein family member Ppa-mbd-2 (ref. 11 ). Ppa-mbd-2(tu365) is recessive, homozygous viable, and displays both a fully penetrant egg-laying defect and a complete absence of the Eu mouth-form ( Fig. 2a ). Ppa-mbd-2(tu365) contains a 1.7 kb deletion that removes four of six exons, suggesting that the absence of the Eu form results from a strong reduction-of-function or even null mutation in this gene. Thus, the phenotype of mbd-2 in P. pacificus reveals the existence of pleiotropic regulators of mouth-form plasticity. 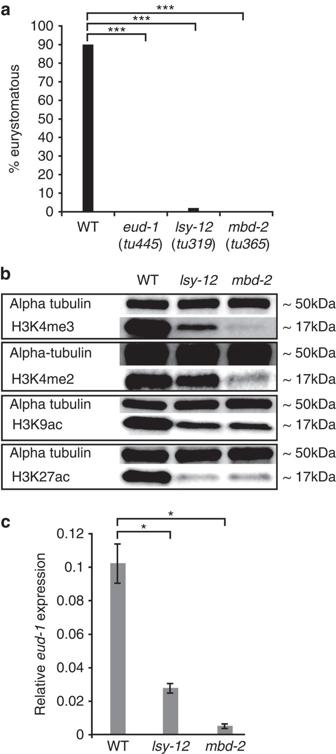Figure 2: Mouth-form defects of two pleiotropic mutants and their effect on histone modification andeud-1expression. (a)Ppa-lsy-12(tu319)andPpa-mbd-2(tu365)result in the (nearly) complete absence of Eu hermaphrodites, similar toeud-1mutants. Data are presented as the total Eu frequency,n>100 for all strains. (b)Ppa-lsy-12andPpa-mbd-2mutants result in severe histone modification defects. This experiment has been replicated three times. (c) qRT–PCR experiments reveal down-regulation ofeud-1expression inPpa-lsy-12andPpa-mbd-2mutants relative to wild type in J2 larvae. This experiment has been replicated three times. Error bars are defined as s.e.m. *P<0.05 and ***P<10−5, Kruskal–Wallis test. Figure 2: Mouth-form defects of two pleiotropic mutants and their effect on histone modification and eud-1 expression. ( a ) Ppa-lsy-12(tu319) and Ppa-mbd-2(tu365) result in the (nearly) complete absence of Eu hermaphrodites, similar to eud-1 mutants. Data are presented as the total Eu frequency, n >100 for all strains. ( b ) Ppa-lsy-12 and Ppa-mbd-2 mutants result in severe histone modification defects. This experiment has been replicated three times. ( c ) qRT–PCR experiments reveal down-regulation of eud-1 expression in Ppa-lsy-12 and Ppa-mbd-2 mutants relative to wild type in J2 larvae. This experiment has been replicated three times. Error bars are defined as s.e.m. * P <0.05 and *** P <10 −5 , Kruskal–Wallis test. Full size image A conserved histone-acetyltransferase regulates plasticity In tu319 mutants, only 2% of hermaphrodites have a Eu mouth-form ( Fig. 2a ). tu319 was isolated in a screen for vulva-defective mutants and represents one of three alleles of the previously genetically characterized vul-2 ( vul valess) locus [12] . Interestingly, only tu319 but not the two other alleles, tu18 and tu30 , show mouth-form defects indicating that the effect of vul-2 on mouth-form regulation is allele-specific. We mapped tu319 to the tip of chromosome IV in proximity to the marker S210 ( Supplementary Fig. 1a ). Sequencing of fosmid clones of this gene poor region resulted in the identification of a histone-acetyltransferase orthologous to the Caenorhabditis elegans gene lsy-12 ( Supplementary Fig. 1b,c ; ref. 13 . Sequencing of lsy-12 identified mutations in all three alleles; tu319 and tu30 have splice-site mutations, whereas tu18 contains a 598 bp deletion in the putative 3′-end of the gene ( Supplementary Fig. 1b ). Ppa-lsy-12 is a complex gene with more than 30 predicted exons, and rapid amplification of cloned/cDNA ends (RACE) and RNA seq experiments provide strong evidence for extensive alternative splicing ( Supplementary Fig. 1b ). Ppa-lsy-12 has a typical MYST domain in the 5′ part of the gene encoded by exons 5–13 ( Supplementary Fig. 1b ), which is present in the majority of transcripts. Interestingly, tu319 affects the splice site of exon 7, whereas the two other alleles affect the 3′ part of the gene, which is not associated with known protein domains and is not present in the majority of transcripts. To attempt phenotypic rescue, we generated a construct of Ppa-lsy-12 containing exons 1–20 (see Methods) and obtained three independently transformed lines carrying the Ppa-lsy-12 construct alongside an egl-20::rfp (red fluorescent protein) reporter. All three transgenic lines rescued both the vulvaless defect and the mouth-form defect of tu319 ( Supplementary Fig. 1c,d ). Specifically, in transgenic animals the mouth-form was 71% Eu (versus 2% Eu in tu319 worms) and, in one line studied in greater detail, 90% of the vulva precursor cells were induced to form vulval tissue (versus 33% in tu319 worms). These results indicate that vul-2 is indeed identical to Ppa-lsy-12 and we renamed the gene accordingly. Taken together, two evolutionarily conserved genes, Ppa-lsy-12 and Ppa-mbd-2 , are pleiotropic regulators of mouth-form plasticity and mutations in these genes result in a strong reduction or absence of the Eu mouth-form. mbd-2 and lsy-12 mutants cause histone modification defects The molecular nature of Ppa-lsy-12 suggests that chromatin remodelling may control the developmental switch mechanism that underlies the P. pacificus mouth dimorphism. Chromatin remodelling proteins regulate numerous developmental processes [14] , but nothing is known of a potential role for chromatin remodelling in the regulation of developmental plasticity. Therefore, we first asked if histone modifications are indeed altered in lsy-12 and mbd-2 mutants. We isolated proteins from mixed stage cultures of wild-type, mbd-2 , and lsy-12 mutant animals and found changes of four histone marks using antibody staining ( Fig. 2b ). H3K4me3 is strongly reduced in both mbd-2 and lsy-12 mutant animals, whereas H3K4me2 is reduced only in mbd-2 mutants ( Fig. 2b ). In contrast, H3K4me1 and several other histone marks are not affected ( Supplementary Fig. 2a ). In addition to H3K4 methylation, the acetylation of H3K27 is strongly, and that of H3K9 moderately, reduced in both mutants ( Fig. 2b ). These findings demonstrate a genome-wide role for MBD-2 and LSY-12 in histone modifications in P. pacificus. Furthermore, because H3K4 methylation and acetylation of various H3 lysines are often found as gene activation marks [14] , these results suggest that the effects of mbd-2 and lsy-12 on mouth-form developmental plasticity is a consequence of chromatin remodelling-mediated transcriptional regulation. eud-1 expression is down-regulated in lsy-12 mutants Next, we tested the developmental switch gene eud-1 as a potential candidate target of chromatin remodelling by LSY-12 and MBD-2. First, we studied eud-1 expression by performing quantitative reverse transcription (qRT)–PCR experiments in wild-type and mutant hermaphrodites in different developmental stages. Indeed, eud-1 is significantly down-regulated in mbd-2 and lsy-12 mutants, in J2 worms, the larval stage at which the mouth-form is determined ( Fig. 2c ). In addition, we also observed eud-1 down-regulation in adult stages, suggesting that eud-1 expression is similarly controlled throughout development ( Supplementary Fig. 2b ). These results suggest that the mouth-form defects of mbd-2 and lsy-12 mutants result from down-regulation of eud-1 . Interestingly, these effects of mbd-2 and lsy-12 mutants on eud-1 expression levels and the mouth-form frequency qualitatively match the patterns seen in P. pacificus males and highly St wild isolates [6] . Altogether, our findings indicate that reduction-of-function or loss-of-function mutations in mbd-2 and lsy-12 cause genome-wide changes in histone modifications, which alter, among other target genes, the expression of eud-1 throughout development. An antisense RNA associated with the eud-1 locus To further explore the function of chromatin remodelling on the regulatory network controlling the developmental switch, we used ultra-directional RNAseq to compare the transcriptomes of wild-type and Ppa-lsy-12 mutant animals ( Fig. 3a ). In total, we found 309 genes to be differentially expressed ( Supplementary Data 1 ). This includes, consistent with our qRT–PCR results eud-1 expression, which was heavily down-regulated in Ppa-lsy-12 worms ( P <10 −8 , Fisher exact test). Surprisingly, however, we also found a strong effect on previously uncharacterized antisense reads at the eud-1 locus ( Fig. 3a ). Indeed, additional RT–PCR experiments identified an antisense eud-1 transcript, termed as- eud-1 . The as- eud-1 RNA consists of three exons with a total size of 863 nucleotides, some of which cover eud-1 exons, such as exons 7–10 and exon 19 ( Fig. 3a ). When we searched for short open reading frames we did not observe any evidence for coding potentials and putative micropeptides longer than 10 amino acids. Thus, as- eud-1 has no obvious open reading frame suggesting that as- eud-1 encodes a long non-coding (lnc) RNA ( Supplementary Fig. 3 ). 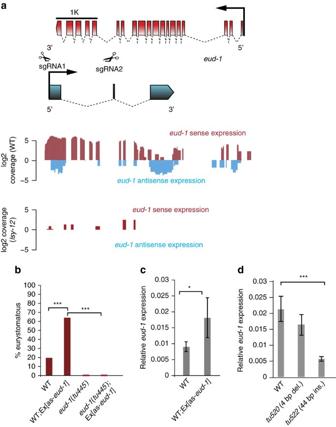Figure 3: Molecular organization and function of as-eud-1. (a) Organization of theeud-1and antisenseeud-1(as-eud-1) locus and RNAseq experiments of wild-type andPpa-lsy-12mutant animals. The long noncoding RNA as-eud-1consists of three exons that span large parts of theeud-1coding region. The structure of as-eud-1was identified in RT–PCR experiments and revealed the existence of a short exon, which went undetected in RNAseq. Other antisense reads obtained at lower frequency in the RNAseq experiment, were not confirmed to be part of as-eud-1in RT–PCR experiments with mixed stage wild-type animals. Subsequent panels show sense and antisense expression as measured for wild-type (wt) andPpa-lsy-12mutant animals. Note that nearly no reads ofeud-1and as-eud-1were observed inPpa-lsy-12mutants. sgRNA1 and sgRNA2 in the 5′ untranslated region (UTR) and exon 2 of as-eud-1, respectively, were used to induce mutations by CRISPR. (b) Transformation of wild-type hermaphrodites with as-eud-1cDNA induced a high incidence of males and a Eud phenotype in male progeny. In contrast, transformation ofeud-1(tu445)mutant animals with as-eud-1did not result in a Eud phenotype, although the high incidence of males was similar to the transformation of wild-type animals. Two independent transgenic lines were generated each,n>100 for all strains. (c) qRT–PCR experiments reveal an up-regulation ofeud-1in as-eud-1transgenic males relative to wild-type males. This experiment has been replicated three times. Error bars are defined as s.e.m. (d) qRT–PCR experiments reveal thateud-1is significantly down-regulated in the as-eud-1promoter mutanttu522that contains a 44 bp insertion. This experiment has been replicated three times. Error bars are defined as s.e.m. *P<0.05 and ***P<10−5, Kruskal–Wallis test. Figure 3: Molecular organization and function of as- eud-1 . ( a ) Organization of the eud-1 and antisense eud-1 (as- eud-1 ) locus and RNAseq experiments of wild-type and Ppa-lsy-12 mutant animals. The long noncoding RNA as- eud-1 consists of three exons that span large parts of the eud-1 coding region. The structure of as- eud-1 was identified in RT–PCR experiments and revealed the existence of a short exon, which went undetected in RNAseq. Other antisense reads obtained at lower frequency in the RNAseq experiment, were not confirmed to be part of as- eud-1 in RT–PCR experiments with mixed stage wild-type animals. Subsequent panels show sense and antisense expression as measured for wild-type (wt) and Ppa-lsy-12 mutant animals. Note that nearly no reads of eud-1 and as- eud-1 were observed in Ppa-lsy-12 mutants. sgRNA1 and sgRNA2 in the 5′ untranslated region (UTR) and exon 2 of as- eud-1 , respectively, were used to induce mutations by CRISPR. ( b ) Transformation of wild-type hermaphrodites with as- eud-1 cDNA induced a high incidence of males and a Eud phenotype in male progeny. In contrast, transformation of eud-1(tu445) mutant animals with as- eud-1 did not result in a Eud phenotype, although the high incidence of males was similar to the transformation of wild-type animals. Two independent transgenic lines were generated each, n >100 for all strains. ( c ) qRT–PCR experiments reveal an up-regulation of eud-1 in as- eud-1 transgenic males relative to wild-type males. This experiment has been replicated three times. Error bars are defined as s.e.m. ( d ) qRT–PCR experiments reveal that eud-1 is significantly down-regulated in the as- eud-1 promoter mutant tu522 that contains a 44 bp insertion. This experiment has been replicated three times. Error bars are defined as s.e.m. * P <0.05 and *** P <10 −5 , Kruskal–Wallis test. Full size image eud-1 and as- eud-1 are co-expressed Next, we tried to determine the expression pattern of as- eud-1 . First, we used various constructs containing a putative 3.5 kb as- eud-1 promoter fragment fused to turbo-RFP but they did not reveal specific expression. Therefore, we established RNA fluorescent in-situ hybridization (FISH) protocols. Indeed, we were able to detect eud-1 RNA in the same head neurons as previously reported for a 7 kb eud-1 promoter fragment driving RFP expression ( Fig. 4a , Supplementary Fig. 4a ; ref. 6 ). FISH of the as- eud-1 RNA and eud-1 RNA revealed that both transcripts are indeed expressed at the same site ( Fig. 4b , Supplementary Fig. 4b ; Supplementary Movie ). Thus, our experiments suggest that eud-1 and as- eud-1 are co-expressed. 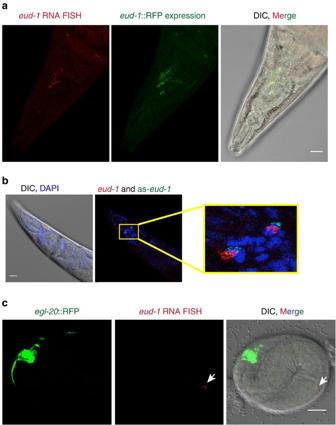Figure 4: Fluorescentin situhybridization (FISH) ofeud-1and as-eud-1reveals co-expression of both transcripts. FISH probes were designed as described in the Methods section. Photographs inaandbshow adult animals, photographs incshow a J1 stage larvae, which inP. pacificusis still in the egg shell. (a)eud-1FISH (red, left image) and aneud-1::RFP reporter construct (green, central image) show the same expression pattern in several head neurons. The image at the right represents a merger of both and differential interference contrast (DIC) microscopy. Note that not alleud-1-expressing cells are visible in this plane of focus. (b) Head area of an adult worm with DIC and 4,6-diamidino-2-phenylindole staining (left image) and co-expression ofeud-1(red) and as-eud-1(green) as revealed by FISH probes. Both transcripts are expressed at multiple foci, two of which are shown in this plane of focus (inset). Overlapping fluorescence (yellow) was seen in all animals observed, but not in all cells. The expression pattern was highly consistent among multiple adults (n>20). SeeSupplementary Moviefor additional details of the partially overlapping expression of both transcripts. (c) Transgenic animals carrying aneud-1::as-eud-1construct showeud-1expression in head neurons already in the J1 stage, which is never seen in wild-type animals.egl-20::RFP (green, left image) is used as transformation marker. The sameeud-1FISH probe (red, central image) was used as above. The image at the right represents a merger and DIC microscopy.Supplementary Fig. 4provides additional photographs foraandb. Scale bars, 10 μm. Figure 4: Fluorescent in situ hybridization (FISH) of eud-1 and as- eud-1 reveals co-expression of both transcripts. FISH probes were designed as described in the Methods section. Photographs in a and b show adult animals, photographs in c show a J1 stage larvae, which in P. pacificus is still in the egg shell. ( a ) eud-1 FISH (red, left image) and an eud-1 ::RFP reporter construct (green, central image) show the same expression pattern in several head neurons. The image at the right represents a merger of both and differential interference contrast (DIC) microscopy. Note that not all eud-1 -expressing cells are visible in this plane of focus. ( b ) Head area of an adult worm with DIC and 4,6-diamidino-2-phenylindole staining (left image) and co-expression of eud-1 (red) and as- eud-1 (green) as revealed by FISH probes. Both transcripts are expressed at multiple foci, two of which are shown in this plane of focus (inset). Overlapping fluorescence (yellow) was seen in all animals observed, but not in all cells. The expression pattern was highly consistent among multiple adults ( n >20). See Supplementary Movie for additional details of the partially overlapping expression of both transcripts. ( c ) Transgenic animals carrying an eud-1 ::as- eud-1 construct show eud-1 expression in head neurons already in the J1 stage, which is never seen in wild-type animals. egl-20 ::RFP (green, left image) is used as transformation marker. The same eud-1 FISH probe (red, central image) was used as above. The image at the right represents a merger and DIC microscopy. Supplementary Fig. 4 provides additional photographs for a and b . Scale bars, 10 μm. Full size image Overexpression of as- eud-1 increases the Eu mouth-form To study the functional significance of this lnc RNA for the mouth-form decision, we performed overexpression experiments of as- eud-1 . Specifically, we generated transgenic animals in which the as- eud-1 complementary DNA (cDNA) is placed under the eud-1 promoter, because the putative as- eud-1 promoter region itself does not drive specific expression of the antisense transcript (see above). Given that eud-1 and as- eud-1 are co-expressed the use of the eud-1 promoter presumably results in overexpression of as- eud-1 . We generated transgenic animals in a wild-type background in order to be able to score the potential effects of as- eud-1 . We obtained three independent transgenic lines, all of which showed a strong masculinization phenotype resulting in more than 95% of animals being males. These transgenic lines showed no embryonic lethality and transgenic males were successfully mated indicating that the high incidence of males result from as- eud-1 -induced X chromosome-specific non-disjunction, a phenomenon known from various C. elegans mutants such as him-8 (ref. 15 ). We, therefore, used the male mouth-form frequency to study the influence of as- eud-1 . In contrast to hermaphrodites, spontaneous wild-type males are only 10–20% Eu because eud-1 is X-linked and dosage-sensitive ( Fig. 1e ; refs 6 , 10 ). The male mouth-form phenotype should be shifted towards more St animals in case of a negative effect and towards higher Eu frequencies in case of a positive function of the as- eud-1 RNA. We made the remarkable finding that as- eud-1 has a positive function on the Eu versus St mouth-form decision and eud-1 expression ( Fig. 3b,c ), whereas most cases of antisense-mediated regulation results in transcriptional down-regulation [16] . Four observations result in this conclusion. First, the frequency of the eud-1 -sensitive mouth-form was dramatically increased in transgenic lines carrying as- eud-1 in a wild-type background (from 20 to 64% Eu males) ( Fig. 3b ). Second, qRT–PCR experiments revealed a strong up-regulation of eud-1 in as- eud-1 transgenic males ( Fig. 3c ). Third, eud-1 RNA can be detected in the J1 stage in eud-1 ::as- eud-1 transgenic animals, an early expression that is never seen in wild-type animals ( Fig. 4c ). Finally, as- eud-1 transgenes in a eud-1 mutant background also caused a high incidence of males, but without affecting male mouth-form. Specifically, eud-1(tu445) ;Ex(as- eud-1 ) males were completely St ( Fig. 3b ), indicating that as- eud-1 acts through eud-1 . Taken together, these experiments suggest that chromatin remodelling acts through antisense-mediated up-regulation of eud-1 . Finally, we used the recently developed CRISPR/Cas9 technology in P. pacificus (ref. 17 ) to generate mutations that would specifically affect as- eud-1 , but not eud-1 . Therefore, we targeted the small exon 2 of as- eud-1 , but were unable to generate a deletion/insertion in this 26 bp exon ( Fig. 3a ). In contrast, we succeeded in generating two mutations in the putative promoter of as- eud-1 ( Fig. 3a ). Specifically, tu520 eliminates a 4 bp fragment, whereas tu522 contains a 44 bp insertion. Both mutant lines show a wild-type mouth-form ratio. However, the tu522 mutant shows significantly reduced eud-1 expression as observed by qRT–PCR experiments ( Fig. 3d ). In contrast, qRT–PCR experiments with as- eud-1 failed to reveal transcripts above background level, a phenomenon known from other lnc RNAs [18] . Altogether, these experiments provide further evidence that as- eud-1 up-regulates eud-1 expression and additionally, they suggest that as- eud-1 expression is itself driven by distal regulatory elements that are unaffected in the tu520 and tu522 mutants. Developmental switching represents an appealing concept to link genetic and environmental influences on phenotypically plastic traits. Our studies of the sulfatase eud-1 —its function as a developmental switch, its role in micro- and macroevolutionary divergence and, here its regulation—provide such mechanistic insights. Previous characterization of eud-1 resulted in several surprising findings, that is its recent origin by gene duplication and its epistasis to other factors controlling feeding plasticity [6] . We have now shown that two evolutionarily conserved genes, mbd-2 and lsy-12 , are involved in genome-wide histone modifications that also influence transcription of eud-1 , providing first insight into the molecular mechanisms underlying the regulation of developmental switches. In particular, the involvement of antisense-mediated up-regulation of eud-1 indicates an unexpected complexity and results in three major conclusions. First, our findings demonstrate that the role of eud-1 involves complex regulation of its own transcription. We previously observed that the coding region of eud-1 is subject to strong purifying selection, and our new findings support and extend these conclusions regarding the importance of regulatory versus structural changes. Second, we demonstrate the involvement of chromatin remodelling in the developmental switch mechanism regulating mouth-form plasticity in P. pacificus . We speculate that chromatin remodelling represents a powerful epigenetic mechanism that might link environmental signals to transcriptional regulation of plasticity. Third, we provide evidence for an antisense RNA in up-regulation. Transcriptional surveys of many eukaryotes have uncovered hundreds of noncoding transcripts [19] and though many of these function as transcriptional regulators, most do so as inhibitors. Conversely, antisense-mediated transcriptional activation or maintenance has only rarely been described [18] , [20] . Thus, the example of as- eud-1 regulation of eud-1 reveals complex regulatory mechanisms that can serve as model to link genetic and environmental control of developmental plasticity in future studies. Culture conditions All wild-type worms were P. pacificus reference strain RS2333. All Pristionchus strains were kept on 6-cm plates with nematode growth medium agar and were fed with a lawn of E. coli OP50 grown in 400 μl L-broth. Cultures were maintained at 20 °C. Because the mouth-form ratio is sensitive to unknown environmental factors [6] , all experiments include their own controls for the wild-type Eu frequency. Also, to minimize the potential for laboratory evolution of the trait, a new culture of the California (RS2333) strain was revived annually from a frozen voucher. Phenotype scoring The mouth-form phenotype was scored using the following characters to discriminate between Eu and St individuals, respectively, (i) the presence versus absence of a subventral tooth, (ii) a claw-like versus flint-like or triangular dorsal tooth, and (iii) a wide versus narrow stoma (mouth). Characters (i) and (ii) were discrete, non-overlapping, and sufficient to distinguish the two forms. Apparent intermediates between the two forms were rare (<0.1%) and were not included in counts. Phenotypes could be scored using Zeiss Discovery V.12 stereomicroscopes and were supplemented where necessary with differential interference contrast (DIC) microscopy on a Zeiss Axioskop. Mapping of vul-2(tu319) and mutant identification For genetic mapping, mutants in the California background were crossed to the Washington strain (PS1843). F2 progeny were cloned and screened for two generations to confirm the mutant phenotype and the homozygosity of mutations. Genomic DNA of outcrossed mutant lines was extracted for genetic mapping. Simple-sequence conformation polymorphism markers were tested against 30–40 outcrossed mutant lines and detected as previously described [21] , [22] . vul-2 was mapped to the tip of chromosome IV close to the marker S210. Further mapping localized vul-2 to the bacterial-artificial-chromosome clone BACPP16-M16 and the fosmid subclones 525-J06, 543-P16 and 558-O23. Light shotgun sequencing of these fosmid clones resulted in the identification of Ppa-lsy-12 as candidate gene for vul-2 . To prepare samples for whole-genomic sequencing, DNA was extracted from all three alleles tu18 , tu30 and tu319 and mutations were identified in all three alleles. Alternative splicing of Ppa-lsy-12 Following preparation of mixed-stage RNA libraries for P. pacificus RS2333, coding DNA (cDNA) was amplified by reverse transcription PCR and sequenced. 5′ and 3′ RACE experiments were performed by SMARTer RACE cDNA Amplification Kit following the manufacturer's protocol (Life Technologies). The full list of gene-specific primers that were designed according to the available genomic sequence for Ppa-lsy-12 is provided in Supplementary Table 1 . RNA-sequencing experiments The presence and levels of gene expression were measured by whole-transcriptome sequencing (RNA-Seq) of Ppa-lsy-12(tu319) mutants and P. pacificus wild type. Culture populations were allowed to grow until their food was exhausted, immediately after which the cultures were processed for sequencing. Five mixed-stage plates were washed with 40 ml M9, centrifuged immediately at 1300 g for 4 min, rinsed with 40 ml 0.9% NaCl treated with 40 μl ampicillin and 40 μl chloramphenicol and shaken gently for 2 h, and finally concentrated into a pellet by centrifugation and immediately frozen in liquid nitrogen. NEBNext Ultradirectional RNA Library Kit (Cat # E7420L) was used to prepare libraries. RNA-Seq libraries were sequenced as 2 × 100-bp paired-end reads on an Illumina HiSeq 2000, yielding 30.6 million reads for the wild type and 31.6 million reads for the lsy-12 sample. Raw reads were aligned to the reference genomes of P. pacificus (Hybrid1) ( www.pristionchus.org ), using the software Tophat v.2.0.3 (ref. 23 ). Expression levels were estimated and tested for differential expression using the programs Cufflinks and Cuffdiff v.2.0.1 (ref. 23 ) resulting in 95 significantly differentially expressed genes including eud-1 (FDR corrected P value<0.01). The equivalent test for down-regulation of as- eud-1 was not significant despite no evidence of as- eud-1 expression in Ppa-lsy-12 animals, which is probably due to the reduced statistical power for differential expression detection resulting from the low expression of as- eud-1 even in wild-type animals. qRT–PCR Total RNA from synchronized cultures was isolated using TRIzol (ambion by life technologies). For reverse transcription Superscript II reverse transcriptase (Invitrogen, Cat. No: 18064) was used following the manufacturer's instructions. We used 1 μg total RNA. The qRT–PCR experiments were performed on a LightCycler 480 system; using SybrGreen (Roche Diagnostics) with a reaction set up described elsewhere [24] . To detect eud-1 expression we used VSe13F GATGATCGAGTCACACAGATCCG forward and VSe13R ATGTAGTAGGAGAGTTGAGCAGCG reverse primers. Ppa-cdc-42 and Ppa-Y45F10D.4 were used as reference genes as previously described [25] . PCR efficiencies were determined using external standards on plasmid mini-preparation of cloned PCR-products. Expression levels were analysed by basic relative quantification. We performed 3–6 biological replicates for different experiments. as- eud-1 transcript analysis RNAseq reads of wild-type worms cover the majority of eud-1 exons to a similar extent. In addition, we observed antisense readsat the eud-1 locus that were previously uncharacterized. These antisense reads are expressed at very low levels and cannot be detected in qRT–PCR experiments, which otherwise are used as a standard procedure in P. pacificus (see above). We used many different PCR primer combinations ( Supplementary Table 2 ) in a variety of nested PCR experiments to study which of the antisense reads if any are present in a potential as- eud-1 cDNA. These experiments revealed the existence of one transcript of 863 nucleotides that consists of three exons ( Fig. 3 , Supplementary Fig. 5 ). The two larger exons cover exactly those reads that were most abundantly found in the RNAseq experiment of wild-type worms. However, exon 2 consists of only 26 nucleotides and went unnoticed at the RNAseq level. Similar to noncoding (nc) RNA (ncRNA) in other systems [18] , as- eud-1 is expressed at very low levels. Genetic transformation For phenotypic rescue of vul-2 , the germ line of vul-2(tu319) mutant animals was injected with a 17 kb genomic construct containing exons 1-20 of Ppa-lsy-12 and 4.5 kb of flanking regulatory region (2 ng ul −1 ), the marker Ppa-egl-20 :: TurboRFP (10 ng ul −1 ) and genomic carrier DNA (60 ng ul −1 from the recipient strain [26] . To study the as- eud-1 lnc RNA, we generated a 7.5 kb construct consisting of ∼ 6.5 kb promoter element and the 860 bp cDNA fragment of as- eud-1 . This construct was injected (2 ng ul −1 ) with the Ppa-egl-20 :: TurboRFP (10 ng ul −1 ) marker and genomic carrier DNA (60 ng ul −1 ) of P. pacificus RS2333 and Ppa-eud-1(tu445) , respectively. For all constructs, at least two independent transgenic lines were generated and transgenic animals were scored over multiple generations involving at least 100 transgenic animals per line. Transgenic lines containing the as- eud-1 lnc RNA yielded more than 90% male progeny and all lines were kept at least until the tenth generation. No embryonic lethality was observed in association with these transgenes. Transgenic males were crossed with Ppa-pdl-1 and wild-type hermaphrodites and cross-progeny was readily observed. CRISPR/Cas9 induced mutations To generate CRISPR/Cas9 induced mutations, sgRNAs were co-injected with Cas9 protein [17] . We used the following sites for single-guided (sg) RNAs (sgRNA): sgRNA1: 5′ CAGTTGAAGAACAAAACACACGG 3′. sgRNA2: 5′ GTCGTAATCAAGCTAACAGCTGG 3′. Statistical analyses All phenotypic data show Eu frequency calculated from total individuals screened. Total sample size is illustrated on graphs. Significant differences were tested by Fisher’s exact test. For the expression data we performed Kruskal–Wallis test. All statistical analyses were implemented in the program Statistica v. 9 (Statsoft). Western blotting and antibodies Proteins were extracted from mixed stage cultures. Concentration was determined by Neuhoff’s Dot-Blot assay [24] . Proteins were equally loaded and separated in polyacrylamid gels. Proteins were transferred to polyvinylidene difluoride transfer membrane and incubated overnight with primary antibodies ( Supplementary Table 3 ), and were then incubated for an hour in secondary antibodies (Anti-rabbit IgG, horseradish peroxidase-linked antibody, Cell Signaling Technology, Cat. #7074S and Anti-mouse IgG, horseradish peroxidase-linked antibody, Cell Signaling Technology, Cat. #7076S). For dilution of primary antibodies see Supplementary Table 3 . The secondary antibody was diluted 1:1,000. The detection was done by Bio-Rad Clarity western enhanced chemiluminescent (ECL) substrate using Peqlab FUSION Xpress multi-imaging system. We provide an uncropped scan of the most important blot as Supplementary Fig. 5 . Single molecule RNA FISH Single molecule RNA FISH was performed using a protocol described earlier for C. elegans [25] . Biosearch Technologies Stellaris FISH online platform was used to design and order eud-s and as-eud-1 probes. They were coupled with Quasar 670 and TAMRA fluorescent dyes, respectively. Image acquisition was performed on Leica SP8 confocal system using settings to maximize detection of fluorescent dyes. Image J software was used for Image analysis. Data availability All relevant data, including mutant and transgenic lines, constructs and plasmids are available upon request from the corresponding author [26] . Accession Codes: The RNA-seq data are available at the NCBI sequence read archive under accession codes SRX1609204 , SRX1858662 , SRX1858663 . How to cite this article: Serobyan, V. et al . Chromatin remodelling and antisense-mediated up-regulation of the developmental switch gene eud-1 control predatory feeding plasticity. Nat. Commun. 7:12337 doi: 10.1038/ncomms12337 (2016).